Bacteroides fragilispolysaccharide A is necessary and sufficient for acute activation of intestinal sensory neurons Symbionts or probiotics are known to affect the nervous system. To understand the mechanisms involved, it is important to measure sensory neuron responses and identify molecules responsible for this interaction. Here we test the effects of adding Lactobacillus rhamnosus (JB-1) and Bacteroides fragilis to the epithelium while making voltage recordings from intestinal primary afferent neurons. Sensory responses are recorded within 8 s of applying JB-1 and excitability facilitated within 15 min. Bacteroides fragilis produces similar results, as does its isolated, capsular exopolysaccharide, polysaccharide A. Lipopolysaccharide-free polysaccharide A completely mimics the neuronal effects of the parent organism. Experiments with a mutant Bacteroides fragilis devoid of polysaccharide A shows that polysaccharide A is necessary and sufficient for the neuronal effects. Complex carbohydrates have not been reported before as candidates for such signalling between symbionts and the host. These observations indicate new neuronal targets and invite further study of bacterial carbohydrates as inter-kingdom signalling molecules between beneficial bacteria and sensory neurons. There are increasing data to suggest that probiotics beneficially modulate adult gut motility, neurons and even behaviour in addition to effects upon the neuroendocrine and immune systems [1] , [2] . Yet the effects on intrinsic enteric neurons are largely unexplored. Feeding with certain bacterial species and strains reduces the perception of visceral pain [3] , [4] , [5] , [6] , decreases activity in spinal single afferent fibres [4] and inhibits colorectal distension induced sensitization of dorsal root ganglion neurons [7] . Ingestion of a Lactobacillus rhamnosus strain, 'JB-1', ( [8] and Methods) moderated the intensity of propagated neuronally dependent peristaltic motor complexes [9] . Luminal application of JB-1 in an ex vivo small intestine peristalsis preparation within minutes reduced the amplitudes of contractions [10] . We hypothesised [10] that this acutely alters the excitability of intestinal primary afferent neurons (IPANs) because the bacteria had no effect on slow wave related contractions, which are independent of the enteric nervous system (ENS) [9] , [10] . Ingestion of Saccharomyces boulardii by pigs decreased expression of a calcium binding protein (calbindin) in IPANs [11] . We have suggested that feeding of JB-1 caused inhibition of an intermediate calcium activated K + channel (IK Ca ) current in mouse myenteric IPANs [12] . However, the mechanisms whereby luminal commensal bacteria communicate with the host nervous system remain obscure. While bacteria can synthesize a large array of neuroactive substances including neurotransmitters [13] , [14] , it is unknown if several molecules mediate specific signalling between bacteria and the ENS. We have not identified JB-1 derived molecules that mimic effects of the whole bacteria on peristalsis, although GABA (γ-aminobutyric acid), a neurotransmitter produced by JB-1 and other bacteria [15] were excluded [10] . However, bacterial components such as glycolipids may be important for signalling between some probiotics and host. For example, certain Lactobacillus species in which capsular lipoteichoic acid is absent or D -alanine depleted, switch from being pro- to anti-inflammatory [16] , [17] in vivo and in vitro , and, with respect to visceral pain in rats, to being antinociceptive [18] . There are no published data to suggest that a luminal polysaccharide might mediate acute neural actions of gut microbiota, although lipopolysaccharide (LPS) from pathogenic bacteria activate spinal sensory neurons upon direct exposure [19] . The zwitterionic capsular exopolysaccharide A, from the anaerobic symbiotic Gram-negative gut bacterium, Bacteroides fragilis (BF) could be a candidate. PSA recapitulated the protective effects of the parent bacterium in models of colitis, and had similar immunoregulatory activity in vitro [20] . These observations prompted us to ask if PSA could mimic any effects that BF may have on IPAN function. If such effects occur, a completely new role for complex polysaccharides might become evident. We have tested whether a single epithelial application of JB-1 or BF could evoke sensory responses [21] in IPANs, facilitate their intrinsic excitability and reduce the 1-[(2-chlorophenyl)diphenylmethyl]-1H-pyrazole (TRAM-34)-sensitive post action potential (AP) slow afterhyperpolarisation (sAHP) that modulates AP accommodation [12] . The sAHP is generated by the opening of an IK Ca channel. As inhibition of an IK Ca channel or its genetic ablation ameliorates T-cell-dependent murine colitis [22] , the bacteria might have therapeutic potential as oral delivery and solubility of the IK Ca channel blocker TRAM-34 are problematic [23] . Indeed, the observation that JB-1 actually does protect against experimentally induced mouse colitis [24] supports this possibility. We devised an ex vivo , hemidissected mucosa myenteric plexus preparation. This combines published in situ mouse myenteric plexus (MP) patch clamp recording methods [25] with our original hemidissection technique of opened intact jejunal segments [21] . The preparation has two separately perfused but contiguous compartments; one with exposed MP and the other, undissected, with intact mucosal epithelium uppermost ( Fig. 1a ). Recordings were made from the MP, and bacteria and test samples added to the epithelial compartment. We were able to test for the first time, whether luminal bacteria or a membrane component can acutely affect sensory neurons, measure the time course of this effect, and make deductions about the cellular mechanisms involved. It has further allowed us to test if a capsular carbohydrate can mimic the signalling and determine it is uniquely responsible for such or part of a more complex possibly plurichemical process. 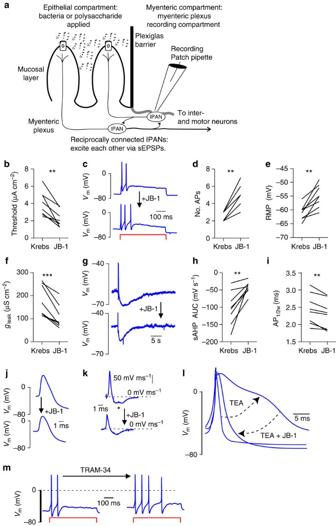Figure 1: Hemidissection preparation and responses of IPANs to adding JB-1 or TRAM-34 to epithelial and myenteric compartments. (a) Patch clamp recordings were made from IPANs (AH cells) in the myenteric compartment; control Krebs or bacteria are applied to epithelium in a separately perfused compartment positioned circumferentially from the myenteric compartment. (b) Firing thresholds decreased after adding JB-1 (**P=0.008, paired-Student’st-test). (c,d) Number of APs fired during test current pulse was increased by JB-1, in example recording (c) upper to lower trace and (d) summary data (**P=0.01, Wilcoxon matched-pairs test). (e,f) JB-1 depolarized IPANs (**P=0.01, paired-Student’st-test) and decreased leak conductances (***P=0.001, paired-Student’st-test). (g,h) Post-AP sAHP was reduced by JB-1, example trace in (g) and summary in (h) (**P=0.008, paired-Student’st-test). (i) JB-1 reduced AP1/2w(**P=0.008, paired-Student’st-test) and this AP narrowing was accompanied by a decrease in the AP hump (j) or inflection (*) on the AP time derivative (k). (l) Adding 10 mM TEA.Cl to the myenteric compartment widened the AP and the hump; subsequent addition of JB-1 to the epithelial compartment significantly reversed the action of TEA (n=5). (m) IPAN exposed to TRAM-34 for 12 min increased the number of APs discharged during a 500-ms test stimulus. The depolarizing stimulus current pulse intensity was 2 × the initial threshold, which was 40 pA for this neuron. Figure 1: Hemidissection preparation and responses of IPANs to adding JB-1 or TRAM-34 to epithelial and myenteric compartments. ( a ) Patch clamp recordings were made from IPANs (AH cells) in the myenteric compartment; control Krebs or bacteria are applied to epithelium in a separately perfused compartment positioned circumferentially from the myenteric compartment. ( b ) Firing thresholds decreased after adding JB-1 (** P =0.008, paired-Student’s t -test). ( c , d ) Number of APs fired during test current pulse was increased by JB-1, in example recording ( c ) upper to lower trace and ( d ) summary data (** P =0.01, Wilcoxon matched-pairs test). ( e , f ) JB-1 depolarized IPANs (** P =0.01, paired-Student’s t -test) and decreased leak conductances (*** P =0.001, paired-Student’s t -test). ( g , h ) Post-AP sAHP was reduced by JB-1, example trace in ( g ) and summary in ( h ) (** P =0.008, paired-Student’s t -test). ( i ) JB-1 reduced AP 1/2w (** P =0.008, paired-Student’s t -test) and this AP narrowing was accompanied by a decrease in the AP hump ( j ) or inflection (*) on the AP time derivative ( k ). ( l ) Adding 10 mM TEA.Cl to the myenteric compartment widened the AP and the hump; subsequent addition of JB-1 to the epithelial compartment significantly reversed the action of TEA ( n =5). ( m ) IPAN exposed to TRAM-34 for 12 min increased the number of APs discharged during a 500-ms test stimulus. The depolarizing stimulus current pulse intensity was 2 × the initial threshold, which was 40 pA for this neuron. Full size image Short latency orthodromic responses to the bacteria and PSA Certain luminal molecules cause IPAN terminals to be activated via mucosal enteroendocrine cells, which release transmitters that stimulate bursts [26] of axonal APs in terminals. These APs then conduct orthodromically from the epithelium to sensory neuron cell bodies, where they can be recorded in the MP [21] . To test if commensal bacteria could similarly activate IPANs, whole-cell patch clamp recordings were made before, during and after a brief (1 s) puff of bacteria or PSA was delivered to the mucosal epithelium abutting the barrier separating the two compartments ( Fig. 1 ). Tested IPANs were always circumferentially opposite the epithelial locus being puffed (as illustrated in Fig. 1 in [21] ). Puffing 7.7 log c.f.u. ml −1 JB-1, BF or 160 ng ml −1 , PSA (see below and Supplementary Methods ) evoked brief low-frequency bursts of orthodromic APs ( Fig. 2 ). These arose directly from resting membrane potential (RMP) baseline without any associated depolarization as seen for synaptic IPAN responses [27] . sAHPs, which are greatly diminished during IPAN synaptic input, were still present, and in some cases proximal process potentials were seen as the membrane hyperpolarised during the sAHP. Furthermore, the AP hump was preserved ( Fig. 2g ) but this was not the case when intrinsic excitability was heightened and ( Fig. 2a ). Onset latencies for the first AP after the beginning of bacteria or PSA application were 8.3±3.3 s (JB-1), n =6, 5.1±3.7 s, n =6 (BF) and 4.9±1.1 s, n =5 (PSA); the AP response frequencies were 1.5±1.1 Hz, n =6 (JB-1) 3.3±2.3 Hz, n =6 (BF) and 5.2±2.8 Hz, n =4 (PSA) ( Fig. 2i ). For 7/17 of the neurons, intrinsic excitability was increased 1 min after the puff ( Fig. 2c versus a ). 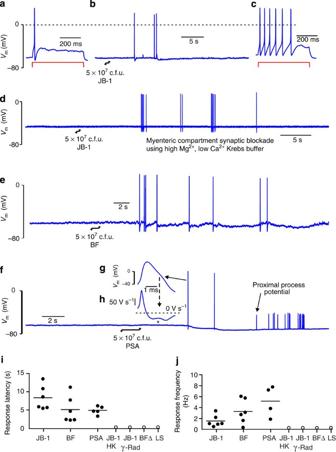Figure 2: Bacteria and PSA that facilitated IPAN intrinsic excitability evoked short latency orthodromic APs. (a) With mucosa exposed to Krebs the IPAN fired only once when a 2 × threshold 500 ms duration current was injected via the recording patch pipette. (b) One second ejection of JB-1 onto the epithelium evoked a short latency burst in IPAN whose intrinsic excitability (c) was increased 1 min later for a second 2 × threshold intracellular current stimulus. (d) Orthodromic response to JB-1 during total synaptic blockade in myenteric chamber (e,f)B. fragilisand its capsular PSA also evoked short latency orthodromic APs in response to their brief application to the epithelium. (g,h) Short latency orthodromic APs retained their characteristic hump and inflection (*) in the differentiated trace. (i,j) Summary statistics for orthodromic responses. JB-1,B. fragilisand PSA, all of which increase IPANs intrinsic excitability, evoked short latency low-frequency IPAN spike bursts when they were puffed onto the epithelium. Heat-killed JB-1 (HK) (n=7), γ-irradiated JB-1 (γ-Rad) (n=6), BFΔ (n=6), or LS (n=6), failed to evoke orthodromic responses. Horizontal lines on scatter graphs indicate means. Figure 2: Bacteria and PSA that facilitated IPAN intrinsic excitability evoked short latency orthodromic APs. ( a ) With mucosa exposed to Krebs the IPAN fired only once when a 2 × threshold 500 ms duration current was injected via the recording patch pipette. ( b ) One second ejection of JB-1 onto the epithelium evoked a short latency burst in IPAN whose intrinsic excitability ( c ) was increased 1 min later for a second 2 × threshold intracellular current stimulus. ( d ) Orthodromic response to JB-1 during total synaptic blockade in myenteric chamber ( e , f ) B. fragilis and its capsular PSA also evoked short latency orthodromic APs in response to their brief application to the epithelium. ( g , h ) Short latency orthodromic APs retained their characteristic hump and inflection (*) in the differentiated trace. ( i , j ) Summary statistics for orthodromic responses. JB-1, B. fragilis and PSA, all of which increase IPANs intrinsic excitability, evoked short latency low-frequency IPAN spike bursts when they were puffed onto the epithelium. Heat-killed JB-1 (HK) ( n =7), γ-irradiated JB-1 (γ-Rad) ( n =6), BFΔ ( n =6), or LS (n=6), failed to evoke orthodromic responses. Horizontal lines on scatter graphs indicate means. Full size image Orthodromic responses were shown to be primary afferent (sensory) rather than trans -synaptic, originating from spinal or vagal sensory terminals. When JB-1 was applied to the epithelium ( n =6) and all synaptic transmission blocked in the myenteric chamber by perfusing the latter with Krebs containing 10 mM MgCl 2 and 0.25 mM CaCl 2 (refs 21 , 27 ), the orthodromic responses persisted ( Fig. 2d ). Consistent with the reduction in extracellular [Ca 2+ ], the calcium-dependent sAHP was abolished ( Fig. 2d ). Negative controls for sensory responses evoked by JB-1 or BF Killed JB-1 or live Lactobacillus salivarius (LS) did not alter migrating motor complexes (MMC) of isolated small intestinal segments when applied to the lumen [10] . As MMC require the activity of myenteric IPANs [9] , we predicted that dead JB-1 or LS would not evoke sensory IPAN responses. JB-1 killed by heating to 80 °C or by γ irradiation as in [4] or live LS (7.7 log c.f.u. ml −1 ) all failed to evoke any orthodromic sensory APs when puffed onto the epithelium ( Fig. 2i ). Because during PSA extraction, BF were only heated to 68 °C (ref. 28 ), we did control experiments where PSA was also heated to 80 °C for 30 min; this treatment did not diminish the ability of PSA to evoke orthodromic sensory potentials in IPANs ( Supplementary Fig. S5 ). Prolonged epithelial exposure to JB-1 As the epithelium may have been compromised in the ex vivo preparation due to a lack of blood supply, we tested for the possibility of a loss of epithelial integrity and bacterial translocation. Adding 7.7 log c.f.u. ml −1 carboxyfluorescein labelled JB-1 to the epithelial compartment for 30 min showed that while some bacteria adhered to the epithelial surface, none translocated to the lamina propria ( Supplementary Methods ). Table 1 summarizes results for the prolonged epithelial exposure experiments for all bacteria used. Table 1 Summary of changes to IPAN intrinsic excitability. Full size table IPANs ( n =8) were patch clamped and their intrinsic excitability, AP and passive membrane properties recorded while the epithelium was bathed in Krebs for 20 min. Then the epithelium was exposed to JB-1 (7.7 log c.f.u. ml −1 in Krebs) and electrophysiological properties tested again. JB-1 increased IPAN intrinsic excitability within 15 min ( Fig. 1b–d ). Firing threshold decreased from 4.0±1.4 to 2.2±1.0 (mean±s.d.) μA cm −2 ( P =0.008, paired-Student’s t -test) and the number of APs discharged during injection of a standard 500 ms current pulse [12] at double threshold intensity increased from 2.4±0.5 to 4.8±1.2 ( P =0.01, Wilcoxon matched-pairs test). These changes were accompanied by a moderate increase in RMP from −61±3 to −55±4mV ( P =0.01, paired-Student’s t -test) ( Fig. 1e ) and a decrease in leak conductance ( g leak ) from 176±52 to 107±68 μS cm −2 ( P =0.001, paired-Student’s t -test) ( Fig. 1f ). The sAHP was diminished by a decrease in absolute area under the voltage–time curve (AUC) from −102±49 to −42±18 mV s −1 ( P =0.008, paired-Student’s t -test) ( Fig. 1g ). Concurrently, AP width at half peak amplitude (AP 1/2w ) narrowed from 2.5±0.4 to 2.3±0.4 ms ( P =0.008, paired-Student’s t -test) ( Fig. 1i ). AP 1/2w narrowing was matched by a reduction in the hump on the AP relaxation phase ( Fig. 1j ). The hump, which can be visualized as an inflection in the AP time derivative (* in Fig. 1k ), was also reduced by JB-1. These changes plateaued 14–20 min after exposure to JB-1. They did not completely washout for at least 30 min after switching back to Krebs. The AP hump, which in IPANs is predominantly caused by the opening of N-Ca 2+ channels [29] , is normally offset by TEA-sensitive potassium conductances that contribute to AP repolarization. We thus unmasked the Ca 2+ dependent hump by adding 10 mM TEA.Cl to the myenteric compartment superfusate [29] . TEA widened AP and emphasized the hump within 5 min of continuous perfusion and this effect was greatly mitigated by a further 10 min perfusion with TEA containing Krebs to which JB-1 was added ( n =5) ( Fig. 1l ). The AP duration was not altered when the AP amplitude was reduced by the decreasing active Na + conductance ( Supplementary Fig. S1d versus f ). These results indicate that JB-1 limits the inward Ca 2+ current during the AP, which in turn would reduce the post-AP IK Ca current, thus reducing sAHP. Effects did not reverse during a 30-min washout period with Krebs [10] . The reduction in IK Ca conductance, which has a constitutive component, is consistent with the observed depolarization as the RMP did not move further away from the potassium equilibrium potential [30] . Brief bursts of APs (such as those evoked by the bacteria) in a single IPAN, signal to neighbouring ones by slow G-protein-dependent metabotropic synaptic transmission. To study if this mechanism had a role in the probiotic action, we tested the effects of the G-protein inhibitor GDPβS on JB-1 induced increase in excitability. JB-1 was added to the epithelial compartment for six experiments and IPANs were patched with electrodes containing GDPβS. For these experiments, JB-1 was now without effect on the sAHP AUC or number of APs evoked at twice stimulus threshold current ( Supplementary Information Fig. S4 ). Blockade of IK Ca mimics the effect on excitability of JB-1 The sAHP is generated by the opening of TRAM-34-sensitive IKCa channels and the resulting hyperpolarisation is limited by a cationic hyperpolarising activated current ( I h ). However, I h was not altered by JB-1 (or BF or PSA) ( Supplementary Information Fig. S3 ) leaving the TRAM-34-sensitive IK Ca as the alternative to explain the observed reductions in sAHP. TRAM-34 (5 μM) ( n =6), which specifically inhibits IPAN IK Ca [9] , [10] , [31] , [32] increased the number of APs fired during a test stimulus at twice threshold intensity from 1.5±0.5 to 4.7±0.8 ( P =0.03, Wilcoxon matched-pairs test) ( Fig. 1m ). Concurrently, the AP firing threshold decreased from 5.6±1.1to 2.6±1.3 μA cm −2 ( P =0.001, paired-Student’s t -test). RMP, g leak and sAHP AUC decreased; 61±3 to 53±2 ( P =0.001, paired-Student’s t -test), 181±18 to 82±25 μS cm −2 ( P =0.0001) and −121±14 to −38±17 mV s −1 ( P =0.0001, paired-Student’s t -test). AP 1/2w was unaffected, 2.3±0.2 versus 2.3±0.2 ms ( P =0.8, paired-Student’s t -test). Negative controls for JB-1 or BF-induced excitability Killed JB-1 or live LS failed to evoke sensory responses (see earlier). Brief sensory AP volleys in IPANs can cause the reciprocally connected slow excitatory IPAN to IPAN network to be activated (see Fig. 4 in [33] ). We predicted that bacteria that fail to induce sensory activation would also not evoke slow postsynaptic excitation within the IPAN network. IPAN excitability was not changed by heat-killed or γ-irradiated JB-1, or live LS (7.7 log c.f.u. ml −1 of each versus luminal Krebs). AP firing thresholds were: 6.1±3.2 versus 6.0±3.0 ( P =0.9, n =8, paired-Student’s t -test), 5.6±1.7 versus 5.4±1.0 ( P =0.8, n =7, paired-Student’s t -test) and 4.8±0.82 versus 4.7±0.8 ( P =0.8, n =7, paired-Student’s t -test) μA cm −2 respectively. The AP numbers fired at twice threshold were similarly unchanged 1.7±0.9 versus 1.5±0.5 ( P =0.4, n =8, Wilcoxon matched-pairs test), 1.3±0.5 versus 1.4±0.8 ( P =0.8, n =7, Wilcoxon matched-pairs test) and 1.8±0.7 to 1.7±0.8 ( P =1.0, n =7, Wilcoxon matched-pairs test). B. fragilis increases IPAN excitability We repeated the hemidissected mucosa myenteric plexus preparation experiments using BF. Freshly washed 7.7 log c.f.u. ml −1 BF suspended in Krebs, was used to perfuse the epithelial compartment ( n =8). BF decreased AP thresholds from 5.9±2.9 to 3.2±2.5 μA cm −2 ( P= 0.002, paired-Student’s t -test), and AP number at twice threshold increased from 1.6±0.7 to 3.9±2.6 ( P= 0.01, Wilcoxon matched-pairs test) ( Fig. 3a–c ). BF also depolarized the RMP from −62±3 to −53±3 mV ( P =0.01, paired-Student’s t -test) and decreased g leak from 192±83 to 130±65 μS cm −2 ( P= 0.008, paired-Student’s t -test) ( Fig. 3d ). BF moderated sAHP ( Fig. 3f ), sAHP AUC changed from −106±63 to −27±30mV s −1 ( P= 0.008, paired-Student’s t -test). AP 1/2w was reduced from 2.3±0.4 to 1.8±0.3 ms ( P= 0.008, paired-Student’s t -test), and consistent with this, the AP hump and the inflection (*) in the AP time derivative were also diminished ( Fig. 3h–j ). 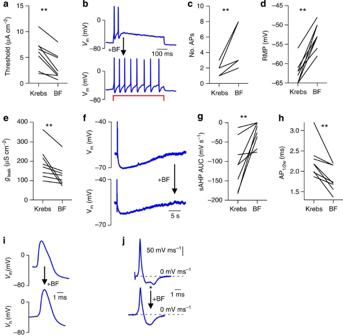Figure 3: Responses of IPANs to adding 7.7 log c.f.u. ml−1BF to epithelial compartment. (a) BF application (n=8) decreased firing thresholds (**P=0.002, paired-Student’st-test), and increased the number of APs fired at 2 × threshold (**P=0.01, Wilcoxon matched-pairs test). (b,c) Example trace and summary data. (d) BF depolarized RMP (**P=0.01, paired-Student’st-test) and (e) decreased leak conductance (P=0.008, paired-Student’st-test). (f,g) BF decreased sAHP (f) example trace and (g) summary data sAHP AUC (**P=0.008, paired-Student’st-test). (h–j) BF narrowed the AP (**P=0.008, paired-Student’st-test). (h) AP1/2wdecreased; (i) the hump and the (j) inflection (*) on the AP time differential were diminished. Figure 3: Responses of IPANs to adding 7.7 log c.f.u. ml −1 BF to epithelial compartment. ( a ) BF application ( n =8) decreased firing thresholds (** P= 0.002, paired-Student’s t -test), and increased the number of APs fired at 2 × threshold (** P= 0.01, Wilcoxon matched-pairs test). ( b , c ) Example trace and summary data. ( d ) BF depolarized RMP (** P =0.01, paired-Student’s t -test) and ( e ) decreased leak conductance ( P= 0.008, paired-Student’s t -test). ( f , g ) BF decreased sAHP ( f ) example trace and ( g ) summary data sAHP AUC (** P= 0.008, paired-Student’s t -test). ( h – j ) BF narrowed the AP (** P= 0.008, paired-Student’s t -test). ( h ) AP 1/2w decreased; ( i ) the hump and the ( j ) inflection (*) on the AP time differential were diminished. Full size image Purified PSA devoid of LPS (see Supplementary Methods ) was initially added at different concentrations to determine IC 50 for effects on sAHP AUC and g leak because the IK Ca current contributes to both parameters [25] , [32] . PSA was added to Krebs perfusing the epithelial compartment at concentrations ranging from 30 ng ml −1 to 1.7 μg ml −1 and concentration response effects were observed. IC 50 for sAHP AUC was −7.0±0.4 log g ml −1 ( n= 28), and IC 50 for g leak was −6.7±0.5 log g ml −1 ( n= 28) ( Fig. 4a ). Additional before–after experiments were performed for six IPANs where 160 ng ml −1 PSA in Krebs was added after control recordings in only Krebs. AP threshold decreased from 6.4±1.4 to 2.7±1.2 μA cm −2 ( P= 0.03, paired-Student’s t -test) and the AP number fired at twice threshold increased from 2.0±0.9 to 9.5±5.2 ( P= 0.03, Wilcoxon matched-pairs test) ( Fig. 4c–e ). RMP depolarized from −60±3 to −49±1 mV ( P= 0.03, paired-Student’s t -test) and the leak conductance decreased from 163±50 to 107±16 μS cm −2 ( P =0.03, paired-Student’s t -test) ( Fig. 4f ). sAHP AUC changed from −120±57 to −39±32 mV s −1 ( P= 0.03, paired-Student’s t -test) ( Fig. 4h ). APs were narrowed by PSA with AP 1/2w from 2.3±0.3 to 1.9±0.3 ms ( P= 0.03, paired-Student’s t -test), and the AP hump was decreased for all six IPANs ( Fig. 4j–l ). These effects plateaued within 4–8 min of applying PSA to the epithelial chamber, after which they persisted without increasing further, and did not washout with normal Krebs for up to 30 min. Congruent with the orthodromic responses, heating PSA to 80 °C did not block its ability to increase IPAN excitability ( Supplementary Fig. S5 ). 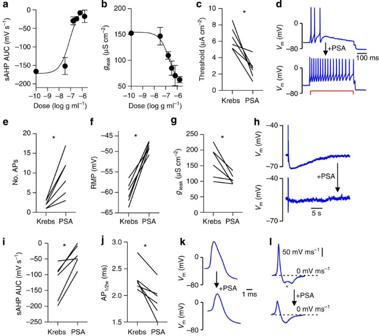Figure 4: IPAN responses to applying PSA to mucosal epithelium. (a,b) PSA concentration response plots (means±s.e.) were fitted with a logistic equation55, IC50for sAHP AUC andgleakwere −7.0 and −6.7 log g ml−1respectively (n=28). (c) PSA (160 ng ml−1) decreased AP firing threshold (*P=0.03, paired-Student’st-test) and (d,e) increased the number of APs fired at twice threshold (P=0.03, Wilcoxon matched-pairs test). (f,g) RMP was depolarized (*P=0.03, paired-Student’st-test) andgleakdecreased (*P=0.03, paired-Student’st-test) by PSA. (h,i) PSA decreased sAHP (h) as measured by absolute AUC (i); also, AP1/2wdecreased (j) and the AP hump (k) and (l) the inflection (*) in the AP time derivative was reduced. Figure 4: IPAN responses to applying PSA to mucosal epithelium. ( a , b ) PSA concentration response plots (means±s.e.) were fitted with a logistic equation [55] , IC 50 for sAHP AUC and g leak were −7.0 and −6.7 log g ml −1 respectively ( n =28). ( c ) PSA (160 ng ml −1 ) decreased AP firing threshold (* P= 0.03, paired-Student’s t -test) and ( d , e ) increased the number of APs fired at twice threshold ( P= 0.03, Wilcoxon matched-pairs test). ( f , g ) RMP was depolarized (* P= 0.03, paired-Student’s t -test) and g leak decreased (* P =0.03, paired-Student’s t -test) by PSA. ( h , i ) PSA decreased sAHP ( h ) as measured by absolute AUC ( i ); also, AP 1/2w decreased ( j ) and the AP hump ( k ) and ( l ) the inflection (*) in the AP time derivative was reduced. Full size image PSA is necessary for the excitatory effects When the epithelial compartment superfusate was changed from Krebs to Krebs containing 7.7 log c.f.u. ml −1 BFΔ for n =10 neurons, AP thresholds were 5.0±1.1 versus 4.8±1.0 μA cm −2 ( P =0.5, paired-Student’s t -test) and the number of AP fired at twice threshold were 3.1±1.9 versus 2.7±1.1 ( P =0.5, Wilcoxon matched-pairs test) ( Fig. 5a ). RMPs were −55±10 versus −58±5 mV ( P =0.08, paired-Student’s t -test), while g leak were 201±41 versus 210±65 μS cm −2 ( P =0.7, paired-Student’s t -test) ( Fig. 5c ). sAHP AUC were −110±68 versus −74±60 mV s −1 ( P =0.08, paired-Student’s t -test) and AP 1/2w were 2.3±0.5 versus 2.0±0.3 ( P =0.1, paired-Student’s t -test) ( Fig. 5e ). These results confirm that the neuronal effects seen with live BF were dependent on the presence of PSA. 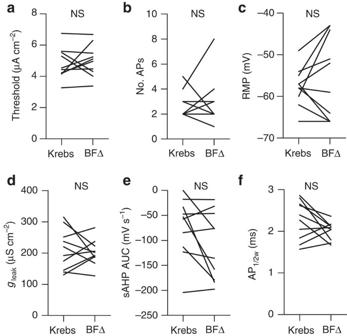Figure 5: BFΔ that lacks PSA when applied to the epithelium did not alter IPAN excitability. (a,b) AP firing threshold (P=0.5, paired-Student’st-test) and number of APs (P=0.5, Wilcoxon matched-pairs test) discharged at twice threshold appeared unaltered by BFΔ. (c,d) BFΔ did not change IPAN RMP (P=0.08, paired-Student’st-test) orgleak(P=0.7, paired-Student’st-test); nor (e,f) were the sAHP AUC (P=0.1, paired-Student’st-test), paired-Student’st-test) or AP1/2w(P=0.1, paired-Student’st-test) altered. Figure 5: BFΔ that lacks PSA when applied to the epithelium did not alter IPAN excitability. ( a , b ) AP firing threshold ( P =0.5, paired-Student’s t -test) and number of APs ( P =0.5, Wilcoxon matched-pairs test) discharged at twice threshold appeared unaltered by BFΔ. ( c , d ) BFΔ did not change IPAN RMP ( P =0.08, paired-Student’s t -test) or g leak ( P =0.7, paired-Student’s t -test); nor ( e , f ) were the sAHP AUC ( P =0.1, paired-Student’s t -test), paired-Student’s t -test) or AP 1/2w ( P =0.1, paired-Student’s t -test) altered. Full size image Epithelial chamber AP propogation underlies excitability We first established that the inter-compartment barrier did not allow tetrodotoxin (TTX) to pass from epithelial to myenteric compartments ( Supplementary Information Fig. 1 ). Neither JB-1 nor BF altered IPAN excitability when AP generation was blocked using TTX in the epithelial chamber. Excitability was measured from 14 IPANs with only normal Krebs in the epithelial compartment, then 0.3 μM TTX plus either 7.7 log c.f.u. ml −1 JB-1 ( n =7) or BF ( n =7) were added to that compartment and excitability measured again for each IPAN. AP thresholds were 5.4±1.0 or 4.8±1.2 μA cm −2 ( P= 0.3, paired-Student’s t -test) for Krebs versus TTX+JB-1, and 5.3±1.2 or 4.9±0.8 μA cm −2 ( P= 0.4, paired-Student’s t -test) for Krebs versus TTX+BF. AP numbers at twice threshold were 1.4±0.8 or 2.0±1.0 ( P= 0.2, Wilcoxon matched-pairs test) for Krebs versus TTX+JB-1 and 1.4±0.8 or 2.1±1.1 for Krebs versus TTX+BF ( P =0.2, Wilcoxon matched-pairs test). As blocking AP conduction blocked the increased excitability, the signalling mechanism did not depend on diffusion of molecules of any size from the epithelium to myenteric neurons. Using a novel in situ gut preparation, we have made the first real-time recordings of acute effects of luminal commensal bacteria on IPANs within minutes of application. This allowed us to deduce how a certain symbiont and probiotic bacteria act on the ENS and thereby gut function. As this parallels the timing of effects on motility in ex vivo peristalsis preparations [10] , the actions of beneficial bacteria on intestinal motility are likely due to actions on neurons rather than second-order effects, which depend on initial involvement of the host’s immune or endocrine systems [34] . This is underscored by our observation that killed JB-1 or LS that do not alter ex vivo motility, also failed to alter IPAN excitability, suggesting strain specificity for probiotic neuroactivity. JB-1 or TRAM-34 both reduced sAHP by 61 or 65%, and doubled or tripled the number of APs fired; neither act on muscle [10] . The physiological correlates of these changes correspond to 50 or 65% decrease in peak amplitude of propulsive contractions [10] when the same doses were used. We recorded for the first time, direct primary afferent APs evoked by applying a probiotic to mucosal epithelium. Brief 1 s puffs of JB-1, BF or PSA evoked orthodromic bursts in IPANs. These were not caused by slow or fast synaptic transmission as there was no membrane depolarization and the upstroke of the AP arose directly from the RMP baseline [35] . AH cells mainly receive afferent presynaptic input onto the soma as they lack dendrites to collect postsynaptic signals sufficiently remote from the soma, and depolarization is not evident [27] , [36] . That synaptic input to the soma was not involved, is further supported by the fact that, after the initial AP volley, proximal process potentials were recorded as the sAHP evolved ( Fig. 2e ) [21] , [35] . Sensory response latencies suggest possible analogies in signalling between the commensal bacteria. The axonal conduction time from the epithelium to myenteric cell body is about 3 ms in guinea pig [35] and 2.3±0.5 ms in mice (Wolfgang A. Kunze, unpublished data n =15). Most AP response latencies could have been caused by enteroendocrine cell receptor activation, intracellular transduction, endocrine cell to neurite signalling and the evolution of neurite receptor potentials until threshold was reached. Similar transduction for mucosal chemosensory afferents can range from a few hundred ms for acetate [33] to 10 or 20 s for amino acids [37] , [38] , long-chain fatty acids [39] or glucose [35] . As responses to JB-1 were about 8 s, it is unlikely that it’s inter-kingdom signalling molecule is acetate or low pH but would be consistent with a saccharide, as we have shown for PSA. Repeated AP trains in presynaptic IPANs evoke a slow increase in excitability (sEPSP) in postsynaptic IPANs with a decrease in AP firing accompanied by membrane depolarization. These occur whether the trains are activated by mucosal field stimulation [33] or direct somal current injection [27] . This self-reinforcing excitatory IPAN network regulates motility [30] , [40] , [41] . During slow synaptic transmission to IPANs, a G-protein coupled decrease in constitutive and AP-associated Ca 2+ currents depolarize the membrane potential, decrease leak conductance, narrow the AP, diminish sAHP and increase intrinsic excitability [30] , [42] , [43] . Similar changes were also induced by JB-1, BF or PSA (Results). Addition of GDPβS (G-protein inhibitor) to the MP compartment blocked effects of JB-1 on sAHP and numbers of APs fired ( Supplementary Information, Fig. S4 ). Thus metabotropic excitation of the IPAN network may contribute to the action of probiotics on the gut. Realistic computational models of MMC indicate that sensory stimulation causes a reflexive buildup of excitability in the enteric circuitry over 10–15 min, which is responsible for the eventual slow onset of contractile responses [41] . This is compatible with the observed 10–20 s latency of probiotic or TRAM-34 effects on gut peristalsis [10] , [44] . Consistent with this is that blocking IPAN IK Ca channels and thus the sAHP with TRAM-34 increased the neurons’ intrinsic excitability ( Fig. 1m ). To explain how IPAN excitability was increased, we propose the following: bacteria and PSA evoke TTX-dependent bursts of AP in IPAN processes innervating mucosal epithelium. These are then conducted through circular muscle to the MP where they invade and traverse IPAN somata to invade axons that project to and synapse on other IPANs [45] . Presynaptic IPANs increase the intrinsic excitability of the postsynaptic IPAN via G-protein-dependent metabotropic (sEPSP) synaptic transmission. As indicated in Fig. 1a , the IPAN being recorded received both direct sensory APs and sEPSPs. When AP generation in the epithelial compartment was extinguished by TTX, JB-1 or BF failed to alter IPAN excitability. As TTX did not diffuse to the myenteric compartment ( Supplementary Fig. S1 ), axonal conduction between mucosa and the MP was required for the increased IPAN excitability elicited. APs would conduct the sensory signals orthodromically (that is, in the usual direction) from the region of sensory transduction towards the somata within the MP [46] . We devised experiments to record such orthodromic responses from IPANs in real-time [21] . LS and killed JB-1, which do not alter motility [10] , also failed to activate IPANs consistent with the concept that effects of probiotic on motility require neuronal sensing of bacteria or their products. We tested BF and its PSA because we do not have an available candidate structural component of JB-1 and because BF effects on IPANs are similar to those of JB-1. The fact that a capsular carbohydrate of BF could mimic the neuronal effects of the whole bacterium opens a new window for mechanistic explorations of how symbiotic and probiotic bacteria communicate with the host. We cannot yet know if PSA acts on epithelial cells that in turn release neuromodulators to act on mucosal IPAN terminals (as for neutral acetate [47] ), or if PSA translocates to directly activate possible receptors on the nerve terminals. To test if PSA was necessary, as well as sufficient to evoke the changes evoked by the whole bacterium, we repeated experiments with a mutant strain of BF lacking PSA (BFΔ). These crucial experiments showed that the mutant had lost the neuromodulatory activity of the parent bacteria. BFΔ had no effect in experiments where PSA recapitulated immunological results of the parent BF [20] . The present paper presents the first quantitative experimental evidence for glycan mediated inter-kingdom signalling between beneficial bacteria and the host ENS. Carbohydrates may serve as unique tools to explore novel pathways for such signalling. Our data favour the likelihood that luminal bacteria and their carbohydrate components interact with cells in the epithelium through pattern recognition receptors such as C-type lectin or toll-like receptors, as these are present on epithelial and enterochromaffin cells [48] . In addition, outer membrane vesicles shed by BF have been shown to contain PSA and by themselves reproduce the immunological effects of the intact bacteria and PSA [49] . However, there are no data indicating what molecules might be released to act on IPANs, but candidates include neurotransmitters such as substance P and CGRP, cytokines, serotonin, melatonin and ATP. Further unravelling how epithelial layer cells transduce bacterial signals to local neuronal elements is clearly an important area for future research. The Hemidissected MP Preparation Our preparation ( Fig. 1a ) represents a modification of the in situ MP patch clamp recording technique [25] , which allows it to be combined with a hemidissection of the preparation so that neurons are exposed for only half the area of an opened small intestinal segment [21] . An excised jejunal segment was placed into a Krebs buffer-filled, carbogen bubbled, recording dish. The segment was opened and pinned mucosa up into the dish fine pins [50] . The mucosa, submucosa and circular smooth muscle were removed, leaving full thickness tissue circumferentially away from the dissected MP area [21] . The recording dish was then mounted on a Nikon TE2000 inverted microscope and the tissue continuously superfused with Krebs saline that was gassed with carbogen. A thin (0.3 mm) Plexiglas partition was placed between the mucosa and exposed MPs and two chambers (2 ml each: epithelial or myenteric) formed and independently perfused with room temperature (18–19 °C) carbogenated Krebs (2 ml min −1 ). The seal between the two chambers was enhanced by lightly coating the edges of the partition with vacuum grease. A single myenteric ganglion, <500 μm from the mucosal edge and with internodal connectives running underneath the mucosa, was selected for cleaning. Now, the temperature of the superfusing Krebs buffer in the myenteric chamber was raised to 35 °C and a 50-μm diameter glass pipette containing 0.02% protease type XI (Sigma-Aldrich, Oakville, Canada) dissolved in Krebs was used to deliver the enzyme to the ganglion for 10–15 min. Then, the enzyme was washed off by increasing the perfusion rate in the myenteric chamber to 10 ml min −1 for 5 min. The connective tissue was ablated using a stream of gravity-fed Krebs delivered by a glass pipette, which was moved across the ganglion until the outlines of individual neuron somata were visualized under brightfield illumination [25] , [51] . The neurons were now ready to be patched ( Supplementary Methods ). Epithelial stimulation To measure direct orthodromic responses, 20 μl of 7.7 log c.f.u. ml −1 bacteria or PSA were puffed directly onto the epithelium using a computer-controlled Valvelink 8 drug perfusion system (AutoMate, San Francisco, USA). Puffs were delivered via a blunted 25-gauge stainless steel needle (inside diameter (ID)=0.24 mm, outside diameter (OD)=0.5 mm). The ejection pressure was 50 hPa and pulse duration was 1 s. When we tested the effects of bacteria on IPAN excitability, the epithelial compartment was first perfused with control Krebs buffer and excitability (firing threshold and number of APs discharged at twice threshold), AP parameters and passive membrane properties were recorded in current clamp mode for at least 20 min. Then the epithelium was stimulated by switching the epithelial chamber inflow to a solution containing the bacteria or PSA in Krebs and physiological recordings were repeated 15 min after solutions were switched. Thirty minutes after switching to bacteria, the inflow was switched back to Krebs alone and measurements repeated. It took 1 min, after switching, for the new solution to reach the epithelial chamber. Preliminary experiments indicated that alterations in excitability plateaued within 15–30 min exposure to bacteria. Bacteria Lactobacillus rhamnosus (JB-1) was taken from in-house stock [4] , [7] , [12] . This bacterium was wrongly identified in several previous publications as L. reuteri and has now been confirmed as a L. rhamnosus by whole-genome sequence analysis. An independent laboratory, the Bacteria Collection Laboratory for Microbiology, University of Ghent, Belgium has further confirmed it to be a rhamnosus using DNA fingerprinting by the AFLP technique. This laboratory was unable to assign the L. rhamnosus (JB-1) to any of the seven intra-specific clusters they have previously reported among 118 strains of this species from around the world [52] and specific comparison with L. rhamnosus (GG) has shown significant differences between these bacteria [8] . All journals in which this wrongly ascribed bacterium has been identified have been asked to publish an erratum or corrigendum containing these facts. All bacterial cell numbers were determined optically and viability was always checked by ability to grow after plating on growth medium agar plates. On the day of the experiment, bacterial cells from frozen stocks were thawed and centrifuged at 2000, r.p.m. for 15 min and the pellet suspended in an equal volume of Krebs buffer. Then the suspension was again centrifuged, the cells removed and resuspended in Krebs at the original concentration. Just before use, bacteria were diluted to working concentrations with Krebs buffer. Bacteria were heat-killed by heating to 80 °C for 20 min after which they lost all viability as shown by cultures up to 72 h after plating. All other related methods are as reported previously [4] , [7] , [12] . Live JB-1 were grown from frozen (−80 °C) 1 ml aliquots, which consisted of 9.7 log c.f.u. in Man-Rogosa-Sharpe broth (Difco Laboratories, Sparks, USA) aliquots. BF strain 9343 originally obtained from the American Type Culture Collection and PSA were gifts from Dennis Kasper (Harvard University). The BF mutant devoid of PSA (BFΔ) was obtained from the same source and is the same bacteria previously described [20] . L. salivarius was a gift from the Alimentary Pharmabiotic Centre, University College Cork [5] . For preparation of polysaccharide A (PSA), the BF were grown anaerobically in 16 l of broth media and extracted with hot phenol/water. Then PSA was purified from the aqueous phase as previously described [28] , [53] . PSA structure and purity were assessed by NMR spectroscopy. No contaminating LPS was previously detected by comparison with purified LPS and it’s absence in the PSA preparation was confirmed by lack of activation of toll-like receptor 4 (ref. 54 ). In addition, we performed LPS control experiments to examine if the excitation of IPANs by PSA possibly could still be attributable to LPS. LPS containing Krebs buffer was made by adding known amounts of LPS (Sigma L2637) to nominally pure buffer, which was made using water filtered with a Nanopure Biological System (Cole-Parmer, Montreal, Canada) water resistivity=18.2 MΩ cm −1 . All chemicals in the Krebs were analytical grade. We applied control Krebs or LPS at −10, −9, −7 or −6 log g ml −1 to the epithelium for 20 min, but there were no measurable alterations in IPAN sAHP magnitude, leak conductance, AP thresholds or number of APs discharged at 2 × threshold current injection ( Supplementary Fig. S2 ) so that contamination by LPS as a cause for any observed action of PSA on sensory neurons is virtually ruled out. Statistics Descriptive data were given as mean±s.d. ( n ), where n is the number of experiments. All statistical tests were two-tailed and, except for action number comparisons, performed using the paired-Student’s t -test. As AP numbers were based on a discrete variable, we used the Wilcoxon matched-pairs test for comparisons involving this parameter. Differences were considered statistically significant at P =0.05. For statistical test outcomes as represented in figure labelling, we followed the convention suggested by Graphpad Prism 6: * denotes P ≤0.05; ** P ≤0.01; ***P<0.001; and ns, P >0.05. Error bars in figures are s.e.m. How to cite this article: Mao, Y-K. et al. Bacteroides fragilis polysaccharide A is necessary and sufficient for acute activation of intestinal sensory neurons. Nat. Commun. 4:1465 doi: 10.1038/ncomms2478 (2013).